Fingerprint of rice paddies in spatial–temporal dynamics of atmospheric methane concentration in monsoon Asia Agriculture (e.g., rice paddies) has been considered one of the main emission sources responsible for the sudden rise of atmospheric methane concentration (XCH 4 ) since 2007, but remains debated. Here we use satellite-based rice paddy and XCH 4 data to investigate the spatial–temporal relationships between rice paddy area, rice plant growth, and XCH 4 in monsoon Asia, which accounts for ~87% of the global rice area. We find strong spatial consistencies between rice paddy area and XCH 4 and seasonal consistencies between rice plant growth and XCH 4 . Our results also show a decreasing trend in rice paddy area in monsoon Asia since 2007, which suggests that the change in rice paddy area could not be one of the major drivers for the renewed XCH 4 growth, thus other sources and sinks should be further investigated. Our findings highlight the importance of satellite-based paddy rice datasets in understanding the spatial–temporal dynamics of XCH 4 in monsoon Asia. Atmospheric methane (CH 4 ) concentration has increased substantially since early 2007, after a hiatus during 1999–2006 [1] , [2] , [3] , [4] , [5] ; however, there is no consensus on the possible causes for this observed increase [1] , [2] , [3] , [4] , [5] , [6] , [7] , [8] , [9] , [10] , [11] . Recent studies suggested that biogenic sources may have contributed most to the ongoing increase of CH 4 emission [4] , [5] , [12] , especially the expansion of tropical agriculture [4] , [5] . Rice paddies are an important biogenic and agricultural source of CH 4 emission and have thus attracted renewed attention [4] , [5] , [12] , [13] , especially in monsoon Asia with 87% of the global paddy rice harvested area and 90% of the rice production (according to FAOSTAT in 2017), and ~25–36% of global CH 4 emissions [13] , [14] . Rice paddy CH 4 emissions are predicted to increase by the end of the 21st century due to the enhancement of rice plant productivity from a warmer climate and atmospheric carbon fertilization [15] , and increased rice paddy area driven by an increasing market demand for rice as a food staple [16] . Hence, it is critical to understand the role of rice paddies in the observed spatial distribution, seasonal dynamics, and interannual variation of atmospheric CH 4 concentration. Advanced satellite measurements of column-averaged concentration of CH 4 (XCH 4 ) provide large-scale constraints for CH 4 emission estimates [17] , [18] , [19] and are used to detect surface CH 4 emission hotspots from space [20] , [21] . The Scanning Imaging Absorption Spectrometer for Atmospheric Chartography (SCIAMACHY) obtained from short-wavelength infrared (SWIR) sensors can measure atmospheric CH 4 concentration from a lower altitude down to the surface, which are more indicative of the emissions from the ground [17] , [18] . SCIAMACHY allows us to uncover and identify the relationships between major sources of surface CH 4 emissions and atmospheric CH 4 columns. Satellite data sets for methane production-related variables (e.g., spatial distribution of methane emission sources) could be useful to associate XCH 4 observations to emission sources [22] . Bloom et al. [18] analyzed the roles of wetlands and rice paddies in determining the temporal dynamics and spatial distribution of atmospheric CH 4 concentration based on the correlations between XCH 4 data from SCIAMACHY and water table depth from the Gravity Recovery and Climate Experiment (GRACE) satellite. They found that the observed seasonal variability of XCH 4 matched closely with the fluctuations in wetlands and rice CH 4 emissions over wetland regions, thus explaining 70% of the methane emissions from surface sources. However, the relative contributions of natural wetlands and rice paddies to the seasonal dynamics and spatial distribution of atmospheric CH 4 concentration in different countries cannot be well quantified using coarse-resolution paddy rice maps (1° × 1°) [18] , [23] and water table depth data from GRACE (3° × 3°) [18] . Hayashida et al. [17] combined XCH 4 data from SCIAMACHY with satellite-derived land surface water coverage (LSWC) and normalized difference vegetation index (NDVI) to quantify the contributions of rice cultivation to the spatial distribution and seasonality of XCH 4 over rice paddy areas derived from agricultural statistics in monsoon Asia. Nevertheless, the relationship between rice cultivation and atmospheric CH 4 concentration in rice paddy regions based on the statistical data of rice harvest areas cannot accurately characterize the role of rice paddies in the seasonal fluctuations of XCH 4 . Although numerous measurements and analyses of CH 4 emission from rice paddies at the site scale have been done [24] , [25] , [26] , [27] , the influence of rice paddies on the spatial distribution and seasonal dynamics of atmospheric CH 4 concentration is still poorly understood at the continental scale, in part due to the lack of moderate to high-spatial resolution maps of paddy rice croplands. The accurate spatial and temporal pattern of rice paddies is critical for understanding the contribution of rice paddies to atmospheric CH 4 concentration. Here, we first generate annual maps of rice paddies in continental monsoon Asia at 500 -m spatial resolution over the period of 2000–2015 through analyses of time series images from Moderate Resolution Imaging Spectroradiometer (MODIS) sensor, using the robust paddy rice mapping algorithms, which were well documented in our previous studies [28] , [29] , [30] , [31] . The resultant annual maps of rice paddies show the spatial–temporal changes of rice paddy areas in monsoon Asia during 2000–2015, including the hot spots and interannual trends. Second, we use the annual MODIS-based paddy rice maps during 2000–2015, MODIS-based vegetation indices, and the XCH 4 data from SCIAMACHY on the Environmental Satellite (ENVISAT) and the Thermal and Near Infrared Sensor for Carbon Observation Fourier-Transform Spectrometer (TANSO-FTS) onboard the Greenhouse Gases Observing Satellite (GOSAT), to quantify the role of rice paddies in determining the spatial distribution and seasonal dynamics of atmospheric CH 4 concentration in monsoon Asia. The results show that geographically those regions with relatively larger proportion of rice paddies have high XCH 4 . In those areas dominated by single- or double-paddy rice cropping systems, the seasonal dynamics of XCH 4 also has one or two peaks in a year, corresponding well with the seasonal dynamics of paddy rice growth. Third, we assess the interannual dynamics of rice paddy area and XCH 4 in monsoon Asia. The results show a decreasing trend of rice paddy area and a renewed growth of XCH 4 in monsoon Asia since 2007. Implications of this study include both a broader perspective regarding satellite-based annual maps of rice paddies at moderate-to-high spatial resolutions and the potential and challenges in understanding the spatial–temporal dynamics of XCH 4 in monsoon Asia. Dynamics of rice paddies in monsoon Asia during 2000–2015 We generated the annual paddy rice maps during 2000–2015 and quantified the spatial–temporal changes in rice paddy area in monsoon Asia. 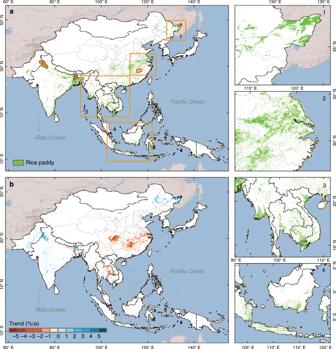Fig. 1: Spatial distributions of paddy rice croplands and its trend from 2000 to 2015 in monsoon Asia. aThe paddy rice map was retrieved from MODIS data with 500 -m resolution in monsoon Asia in 2015.bThe spatial pattern of trends in rice paddy area at 5 × 5 km gridcells during 2000–2015.1–4Detailed spatial distributions of rice paddies in local regions, labeled inawith orange rectangles. The small and red polygons inaare the samples illustrated in Fig.3. Source data are provided as a Source Data file. Figure 1a shows the spatial pattern of rice paddies in 2015 over monsoon Asia at 500 -m spatial resolution. China and India had the largest total area of rice paddies, and together accounted for over half the total rice paddy area in monsoon Asia (Supplementary Fig. 1 ). Rice paddies were mainly located in the alluvial plains of major rivers in this region, including the Indo-Gangetic Plain in eastern India, Yangtze Plain in southern China, Ayeyarwady Delta in southern Myanmar, and Mekong Basin in Southeast Asia. The rice paddies in monsoon Asia substantially increased from 2000 to 2007, but then decreased from 2007 to 2015 (Supplementary Fig. 2 ). Geographically, those regions with significant decreasing trends in rice paddy area during 2000–2015 included the Yangtze Plain of southern China and eastern Thailand, while Northeast China and India had significantly increasing trends in rice paddy area (Fig. 1b ). These annual maps provide improved data and knowledge of the spatial distribution and interannual variation of rice paddy in monsoon Asia. Fig. 1: Spatial distributions of paddy rice croplands and its trend from 2000 to 2015 in monsoon Asia. a The paddy rice map was retrieved from MODIS data with 500 -m resolution in monsoon Asia in 2015. b The spatial pattern of trends in rice paddy area at 5 × 5 km gridcells during 2000–2015. 1 – 4 Detailed spatial distributions of rice paddies in local regions, labeled in a with orange rectangles. The small and red polygons in a are the samples illustrated in Fig. 3 . Source data are provided as a Source Data file. Full size image Spatial consistency between rice paddies and XCH 4 We investigated the relationships between the MODIS-based paddy rice maps and satellite observed XCH 4 in monsoon Asia at various spatial and temporal scales. The spatial distributions of rice paddies were consistent with those of atmospheric CH 4 concentration over six 3-year moving-window periods (2003–2005, 2005–2007, 2007–2009, 2009–2011, 2011–2013, and 2013–2015, Fig. 2a–f ; Supplementary Fig. 3a–f ). Those regions with high densities of rice paddies also had high XCH 4 . For example, the high densities of rice paddies in Indo-Gangetic Plain in north India, Bangladesh, and the Yangtze Plain and Sichuan Basin in China matched closely with those areas with high XCH 4 (Fig. 2a–f ; Supplementary Fig. 3a–f ). Fig. 2: Consistency of spatial distributions between paddy rice croplands and atmospheric methane concentration. The three periods (2003–2005, 2007–2009, and 2011–2013) were selected in the main text to illustrate the spatial relationships between rice paddies and XCH 4 . a – c Spatial distributions of 3-year averaged area proportions of MODIS-based paddy rice croplands for 2003–2005 with 0.5° gridcells ( a ), 2007–2009 with 0.5° gridcells ( b ), and 2011–2013 with 2.0° gridcells ( c ). d – f Spatial distributions of 3-year averaged annual column-averaged concentration of CH 4 (XCH 4 ) from SCIAMACHY for 2003–2005 with 0.5° resolution ( d ), 2007–2009 with 0.5° resolution ( e ), and from TANSO-FTS for 2011–2013 with 2.0° resolution ( f ). g – i 3-year averaged annual XCH 4 for different rice paddy area proportions for 2003–2005 ( g ), 2007–2009 ( h ), and 2011–2013 ( i ). The x -axis values in figures ( g – i ) represent levels of rice paddy area proportions in monsoon Asia, and 1–7 correspond to <0.5%, 0.5–1%, 1–5%, 5–10%, 10–20%, 20–40%, and >40% rice paddy area proportions, respectively. Source data are provided as a Source Data file. Full size image Different densities (% percentage) of rice paddies within individual gridcells over each of the 3-year periods were divided into seven intervals (a gradient), and the XCH 4 within each interval were analyzed. The 3-year mean XCH 4 increased as the density of rice paddies rose for all these 3-year periods (Fig. 2g–i ; Supplementary Fig. 3g–i ). Similar relationships were also found in different seasons in these periods (Supplementary Figs. 4 – 7 ). We used the spatial error model (SEM) to quantify their spatial relationships during the six 3-year periods, and the results showed that the density of rice paddies had high spatial correlation with the 3-year mean XCH 4 ( P -value of coefficients < 0.001, and P -value of Moran’s I test of residuals > 0.3) for all these periods (Supplementary Table 1 ). It should be noted that clouds and shadows in the inter-tropical convergence zone (e.g., Indonesia and Malaysia) occur frequently (Supplementary Fig. 8 ), which could affect satellite-based optical images used for paddy rice mapping and XCH 4 retrieval. In those areas with frequent cloud cover and shadows, there is potentially a multicollinearity issue in the rice paddy area and XCH 4 data. We re-ran the SEM analysis for the other monsoon Asia countries after excluding Indonesia and Malaysia, and the results still showed strong spatial consistency between rice paddy area and XCH 4 (Supplementary Figs. 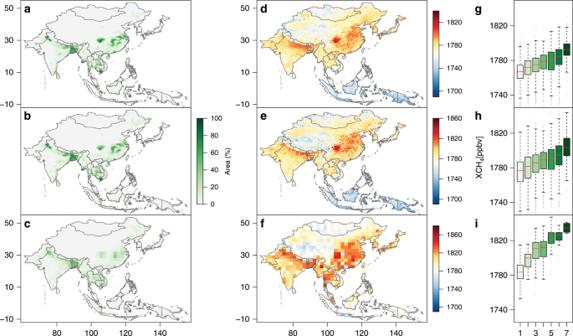Fig. 2: Consistency of spatial distributions between paddy rice croplands and atmospheric methane concentration. The three periods (2003–2005, 2007–2009, and 2011–2013) were selected in the main text to illustrate the spatial relationships between rice paddies and XCH4.a–cSpatial distributions of 3-year averaged area proportions of MODIS-based paddy rice croplands for 2003–2005 with 0.5° gridcells (a), 2007–2009 with 0.5° gridcells (b), and 2011–2013 with 2.0° gridcells (c).d–fSpatial distributions of 3-year averaged annual column-averaged concentration of CH4(XCH4) from SCIAMACHY for 2003–2005 with 0.5° resolution (d), 2007–2009 with 0.5° resolution (e), and from TANSO-FTS for 2011–2013 with 2.0° resolution (f).g–i3-year averaged annual XCH4for different rice paddy area proportions for 2003–2005 (g), 2007–2009 (h), and 2011–2013 (i). Thex-axis values in figures (g–i) represent levels of rice paddy area proportions in monsoon Asia, and 1–7 correspond to <0.5%, 0.5–1%, 1–5%, 5–10%, 10–20%, 20–40%, and >40% rice paddy area proportions, respectively. Source data are provided as a Source Data file. 9 – 12 and Supplementary Table 2 ). These results suggested that the spatial distribution of rice paddies was one of the major factors that determine the spatial distributions of atmospheric CH 4 concentration in monsoon Asia. Seasonal consistency of paddy rice growth and XCH 4 Enhanced vegetation index (EVI) is related to vegetation canopy [32] (Supplementary Fig. 13 ), and has been used to estimate gross primary production of paddy rice [33] . We used MODIS-based EVI as a proxy for rice plant growth to quantify the seasonal relationship between the paddy rice growth and atmospheric CH 4 concentration in a year. We analyzed time series EVI and XCH 4 data at selected regions of interest (ROIs) with different rice cropping systems and rice paddy-dominated regions in monsoon Asia. First, we analyzed the seasonal dynamics of XCH 4 and paddy rice growth in four typical ROIs with a high density of rice paddies and different cropping systems (single- and double-cropping systems) (Fig. 3 ). We calculated mean EVI for all pixels within 0.5° gridcells (EVI all-pixels ), mean EVI for all rice paddy pixels within 0.5° gridcells (EVI all-rice ), and EVI for one rice paddy pixel with 500 -m resolution (EVI rice ). The seasonal dynamics of XCH 4 had one peak per year in three regions (Northeast China, northern India, and northern Bangladesh, Fig. 3e–g ), and two peaks per year in one region (southern China, Fig. 3h ). The consistency in the peak timings of XCH 4 and EVI clearly increased from EVI all-pixels to EVI all-rice and EVI rice , suggesting the contribution of rice growth to XCH 4 . The Sanjiang Plain of Northeast China (Fig. 3a ) had a single crop per year, mostly paddy rice. Remarkably, both XCH 4 (Fig. 3e ) and EVI (Fig. 3i, m, q ) had a single peak around August in each year, and the seasonal dynamics of XCH 4 corresponded well with those of the three EVI data sets (all of Pearson’s correlation coefficients between EVI and XCH 4 during the entire year R year ≥ 0.60, P < 0.001, Fig. 3i, m, q ). Northern India and northern Bangladesh (Fig. 3b, c ) had a double-cropping rotation with winter wheat/rainfed rice and paddy rice in each year according to previous studies [34] , [35] . The seasonality of XCH 4 (Fig. 3f, g ) had only one peak, which corresponded well with the seasonality of paddy rice (the second crop in these regions) in the EVI all-pixel , EVI all-rice , and EVI rice data (Fig. 3 j, k, n, o, r, s , all of the Pearson’s correlation coefficients between EVI and XCH 4 during the summer-fall season from May to November R 5–11 larger than R year ). The Poyang Lake region of southern China (Fig. 3d ) had a mixture of single rice and rice–rice double-cropping rotations in one year [36] . The annual XCH 4 (Fig. 3h ) in this region had two distinct seasonal cycles, which corresponded well with the seasonal dynamics of EVI rice (Fig. 3t ). It should be noted that there were no obvious double peaks for EVI all-pixel and EVI all-rice in one year at a coarse spatial gridcell resolution of 0.5° resolution (Fig. 3l, p ) due to the mixture of single and double rice cropping rotations in this region. These results suggested that the growth cycle of paddy rice contributed significantly to the seasonality of XCH 4 . Fig. 3: Seasonal dynamics of atmospheric methane concentration and rice growth. The column-averaged methane concentration (XCH 4 ) and the enhanced vegetation index (EVI) were analyzed in four regions of interest (ROIs) with dense rice paddies and different cropping systems. a – d Spatial distributions of rice paddies retrieved from MODIS data with 500 -m resolution in the Sanjiang Plain of Northeast China in 2010 with single cropping paddy rice ( a ), North India in 2005 with winter wheat and paddy rice ( b ), North Bangladesh in 2005 with rainfed rice and paddy rice ( c ), and Poyang Lake of China in 2005 with early and late paddy rice ( d ). The four ROIs are shown in Fig. 1a with small and red polygons. e – h Time series of monthly SCIAMACHY CH 4 column volume mixing ratios (VMRs, in parts per billion) over the corresponding four ROIs labeled in ( a – d ) with red polygons. i – l Time series of monthly MODIS-based EVI for all pixels within 0.5° gridcells (EVI all-pixels ) over the aforementioned four ROIs. m – p Time series of 8-day EVI values for all 500 m rice paddy pixels within the 0.5° gridcells (EVI all-rice ). q – t Time series of 8-day EVI values for one rice paddy pixel with 500 m resolution (EVI rice ). The four bottom images are the corresponding landscapes for each rice paddy pixel ( q – t ) with the extent of 500 m by 500 m from Google Earth. R year and R 5–11 offer the Pearson’s correlation coefficients between XCH 4 and EVI for the whole year and summer-fall season from May to November during the corresponding period labeled in the x -axis of ( q – t ). *** P < 0.01; * P < 0.10. Correlation coefficients without asterisk are insignificant ( P > 0.10). Source data are provided as a Source Data file. Full size image It is well recognized that rice plants play a critical role in the processes of methane production [37] , [38] . Several recent in situ studies found a strong correlation between daily CH 4 flux and rice plant biomass, which suggested that methane flux in rice paddies is affected by rice growth and development [37] , [38] , [39] , [40] , [41] , [42] , [43] , [44] . Here, we compared the observed CH 4 emission and EVI at eight paddy rice sites [25] , [26] , [27] , [41] , [42] , [45] , [46] , [47] , and the results confirmed their consistency in terms of seasonality (Supplementary Fig. 14 ). The synchrony of rice growth and CH 4 emissions is due to the fact that the rhizodeposition from current season photosynthesis and plant growth controlled the organic matter of the flooded soils, and subsequently determined the methanogenesis in paddy soils [38] , [48] , [49] . Rice plants provide root exudates, which is the important organic matter used by soil microbes for CH 4 production in rice paddies [37] , [44] . The quantity of root exudates varies during the rice plant growing season, which rises as the rice plants grow, reaches a maximum during the flowering stage with a peak in root biomass, and then decreases (Supplementary Fig. 13 , Supplementary Note 1) [38] . Although this synchronized peak has been previously found at field site, our results using satellite data show synchrony at large scales for the first time with the aid of high-resolution paddy rice maps. Moreover, the rice cropping systems affected the peaks in XCH 4 , that is, the XCH 4 variation was controlled by the paddy rice growth cycle regardless of whether it was a single- or double-cropping system (wheat–rice, rice–rice) (Fig. 3 ). The ROI-scale analyses suggested the modeling of the seasonal dynamics of atmospheric CH 4 concentration need to consider the rice cropping system (single rice, double rice, or rice plus other crop) rather than general cropping intensity (single, double, or multiple cropping). Second, we further analyzed the spatial patterns of seasonal consistency between paddy rice growth and XCH 4 in monsoon Asia using monthly EVI all-rice and XCH 4 at 0.5° gridcells during 2003–2005 (Fig. 4 ). Figure 4a, b showed the spatial patterns of the Pearson’s correlation coefficients between EVI and XCH 4 during the entire year (R year ) and the summer-fall season from May to November (R 5–11 ) during 2003–2005, respectively. 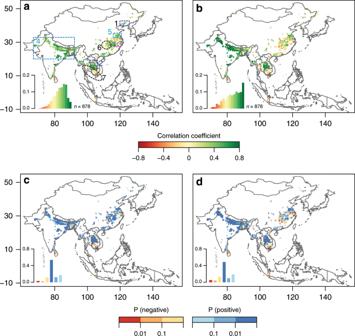Fig. 4: Spatial patterns of correlations between seasonal atmospheric methane concentration and rice growth. The monthly atmospheric column-averaged methane concentration (XCH4) from SCIAMACHY and the enhanced vegetation index (EVI) from MODIS were analyzed in the dense rice paddy areas of monsoon Asia during 2003–2005.a,bThe spatial distributions of Pearson’s correlation coefficients between XCH4and EVI for the whole year and summer-fall season from May to November, respectively.c,dThe spatial distributions of significance levels of Pearson’s correlation between the two for the whole year and summer-fall season from May to November, respectively. The region with a 3-year averaged rice paddy gridcells with area proportion larger than 10% during 2003–2005 is considered here. The insets in (a–d) are the corresponding frequency diagrams of Figure (a–d). Source data are provided as a Source Data file. 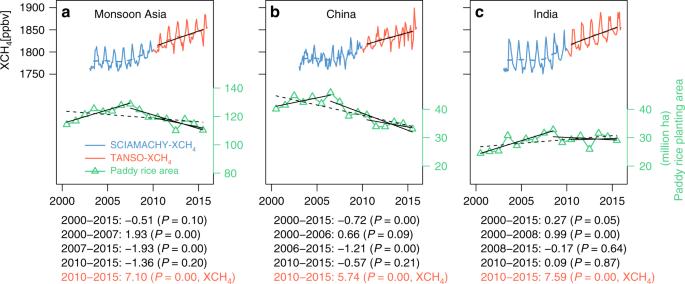Fig. 5: Temporal dynamics of atmospheric methane concentration and rice paddy area. Temporal (seasonal and interannual) dynamics of atmospheric column-averaged methane concentration (XCH4) over rice paddy-dominated regions and interannual variations in MODIS-based rice paddy areas during 2000–2015 in monsoon Asia (a), China (b), and India (c). The curves above are time series of monthly SCIAMACHY CH4column volume mixing ratios (VMRs, in parts per billion) during 2003–2009 and monthly TANSO-FTS CH4column VMRs during 2010–2015. The XCH4outliers in winter have been removed. The blue and red dashed lines are average annual values of SCIAMACHY XCH4and TANSO-FTS XCH4, respectively. The black lines and black dashed lines below indicate trends of rice paddy area for different periods in monsoon Asia, China, and India. The rice paddy-dominated regions are shown in Supplementary Fig.35. The linear trends and its significance levels for different periods are shown below the panels; the formulas in black color are for paddy rice planting area, and the formula in red is for XCH4. Source data are provided as a Source Data file. Regions with the same or similar cropping system and planting schedule demonstrated clear relationships between paddy rice growth and XCH 4 . Most 0.5° gridcells in regions dominated by a single rice crop in a year had statistically significant and positive Pearson’s correlation coefficients between EVI all-rice and XCH 4 at both yearly and seasonal scales (R year and R 5–11 ), as seen in the Liaohe Plain in China [31] (Region 1 in Fig. 4a ) and eastern Thailand [50] , [51] (Region 2 in Fig. 4a , Supplementary Fig. 15 ). Most 0.5° gridcells in regions dominated by double rice cropping systems (rice–rice rotation) also had statistically significant and positive Pearson’s correlation coefficients between EVI all-rice and XCH 4 data at both annual and seasonal scales (R year and R 5–11 ), as seen in southern China [36] (Region 3 in Fig. 4a ); however, the area was small due to the limited double-rice croplands [52] . The 0.5 gridcells in regions with double cropping systems of rice and another crop (e.g., rice and winter wheat) had positive R year and R 5–11 values, but R 5–11 values were obviously larger than R year . These results can be seen in North India and Bangladesh [34] , [35] (Region 4 in Fig. 4a , Supplementary Fig. 15 ), as well as North China [53] (Region 5 in Fig. 4a ). Fig. 4: Spatial patterns of correlations between seasonal atmospheric methane concentration and rice growth. The monthly atmospheric column-averaged methane concentration (XCH 4 ) from SCIAMACHY and the enhanced vegetation index (EVI) from MODIS were analyzed in the dense rice paddy areas of monsoon Asia during 2003–2005. a , b The spatial distributions of Pearson’s correlation coefficients between XCH 4 and EVI for the whole year and summer-fall season from May to November, respectively. c , d The spatial distributions of significance levels of Pearson’s correlation between the two for the whole year and summer-fall season from May to November, respectively. The region with a 3-year averaged rice paddy gridcells with area proportion larger than 10% during 2003–2005 is considered here. The insets in ( a – d ) are the corresponding frequency diagrams of Figure ( a – d ). Source data are provided as a Source Data file. Full size image The relationships between EVI all-rice and XCH 4 data in regions with heterogeneous annual cropping systems and rotation schedules were more complicated and irregular, and the 0.5° gridcells in these regions had non-significant or negative R year and R 5–11 values. Such complexities were observed in the Yangtze Plain in southern China and western Thailand, which had a mixture of single- and double-rice cropping systems [36] , [50] , [51] , [52] , and in Cambodia and southern Vietnam, which had a mixture of single-, double-, and triple-rice cropping systems [50] , [54] (Regions 6 and 7 in Fig. 4a ; Supplementary Fig. 15 ). The two measures most likely failed to positively correlate because EVI and XCH 4 at 0.5° gridcells could be affected by the heterogeneity of cropping systems, crop types, and rice planting schedules, as well as cloud cover. For example, the Mekong Delta of Vietnam has single-, double-, and triple-rice cropping systems that are either rain-fed or irrigated [54] . The EVI and XCH 4 profiles from this region with mixed cropping systems had irregular seasonal patterns and accordingly weak or negative correlations (Supplementary Fig. 16 ), which could also be affected by the uncertainty of observed EVI and XCH 4 due to intensive cloud cover. A similar result was found for the period of 2005–2007, 2007–2009, and 2009–2011 (Supplementary Figs. 17 – 19 ). The significant correlations between EVI and XCH 4 in rice paddy areas with the same or similar cropping systems and planting schedules (Figs. 3 , 4; Supplementary Figs. 17 – 19 ) demonstrated the role of rice paddies in determining the seasonal dynamics of atmospheric CH 4 concentration in monsoon Asia. Our analyses demonstrate that the satellite-observed XCH 4 is indicative of CH 4 emissions from rice paddies, and paddy rice cultivation dominates the spatial distribution and seasonal dynamics of atmospheric CH 4 concentration over those regions with dense rice paddies. This study also shows the importance of annual paddy rice maps for assessing the effects of rice paddies on the spatial pattern and seasonal dynamics of atmospheric CH 4 concentration by providing more details on the location and area proportion within gridcells. On one hand, these maps could show area fractional information within the 0.5° and 2° gridcells when analyzing spatial relationship between rice paddy area and XCH 4 . On the other hand, they allow us to capture the seasonal dynamics of vegetation indices for individual rice paddies (pixels) when analyzing seasonal relationship between them. The temporal statistics of vegetation indices for all pixels within individual gridcells often differ from those for the pure rice paddy pixels (e.g., Fig. 3j, n ). The pure rice paddy pixel-based analyses had clear double peaks (EVI all-rice in Fig. 3n ), while only one peak was found for all the pixels (EVI all-pixels in Fig. 3j ) due to disturbances from other upland crops or natural vegetation types in the gridcells. Although the 500 m paddy rice maps in this study still had mixed pixel issues, this paddy rice product provided unprecedented details on location and area proportion within the 0.5° or 2° gridcells for the entirety of monsoon Asia, in comparison with previous efforts that used county- or province-level paddy rice data [14] , [17] , [55] , [56] . Therefore, it is necessary to use accurate paddy rice maps at moderate spatial resolution as masks to track seasonal fluctuations of atmospheric CH 4 concentration. In addition to the density of rice paddies within gridcells, our results also demonstrate the importance of the information about rice cropping intensity (single or double) and timing of rice crop calendar within gridcells. The seasonal dynamics of XCH 4 , which have one or two peaks in a year, mirror paddy rice growth in the areas dominated by single- and double-rice cropping systems (Fig. 3 ). Together, the accurate information on the locations of rice paddies allow us to fingerprint the effects of rice paddies on atmospheric CH 4 concentration, which can reduce influence from other land cover types in the gridcells. Furthermore, the spatial distribution of rice paddies in monsoon Asia has changed substantially since 2000, including a northward shift of rice paddies in China [30] . Therefore, the methane emission simulations should be conducted with annual maps of rice paddies to more accurately estimate the effects of changing paddy rice distribution on methane emissions since 2000. Interannual dynamics of rice paddy area and XCH 4 Recent increases in atmospheric CH 4 concentration since 2007 are not well understood as evidenced by many hypotheses currently debated [1] , [2] , [3] , [4] , [5] , [6] , [7] , [8] , [9] , [10] , [11] . Some studies reported that biogenic sources, most notably agriculture, may be the key contributor to renewed growth in atmospheric CH 4 [4] , [5] . Rice paddy is one of the main agricultural sources of CH 4 emission. In this study, we also investigated whether interannual variations in rice paddy area contributed to the renewed growth of atmospheric CH 4 concentration since 2007 at the national and continental scales. We analyzed the interannual variations of XCH 4 during 2003–2015 in monsoon Asia, especially China and India, the two countries with the largest rice paddy areas. The interannual variations in XCH 4 in the rice paddy-dominated areas of monsoon Asia, China, and India were relatively stable during 2003–2006, but changed into an increasing trend beginning in 2007 (Fig. 5 ), which agreed well with the trends of global XCH 4 [1] . The rice paddy area increased during 2003–2006 in China, India, and monsoon Asia, but after 2007 rice paddy area decreased in China and monsoon Asia and remained stable in India (Fig. 5 ). The total rice paddy area in monsoon Asia has declined since 2007 over the time period of renewed XCH 4 growth. Similar results were also found for the whole region (rice paddy and non-rice paddy areas) of monsoon Asia, China, and India (Supplementary Fig. 20 ). In theory, if the interannual trends of rice paddy area and the atmospheric CH 4 concentration are consistent, we cannot conclude that rice paddy area is the main driver for the regrowth of atmospheric CH 4 concentration since 2007. If their trends are opposite, we can conclude that the rice paddy area is not the main driver for the regrowth of atmospheric CH 4 concentration. The decreasing trends of rice paddy area and the increasing trends of atmospheric CH 4 concentration in both the rice paddy-dominated areas and the whole area since 2007 suggested that the change in rice paddy area was not the main driver for the renewed increase of atmospheric CH 4 concentration. A study using atmospheric methane observations and an atmospheric transport model reported that the annual methane emission has not significantly changed in India during 2010–2015 and the major CH 4 sources (ruminants, rice paddies, waste, and fossil fuels) did not much change [57] , which is in line with the stable rice paddy areas in India from this study during the same period (Fig. 5 ). Another country-scale study showed that rice paddies did not contribute to the increase of atmospheric CH 4 concentration in China and India during 2010–2015 using the emission estimates from the inverse model and the spatial distribution of different source sectors within the EDGAR emissions inventory [58] , which agrees with our result from 2010–2015 (Fig. 5 ). Our study at monsoon Asia scale suggests that the renewed growth of atmospheric CH 4 concentration was unlikely attributed to the dynamics of rice paddy area. Fig. 5: Temporal dynamics of atmospheric methane concentration and rice paddy area. Temporal (seasonal and interannual) dynamics of atmospheric column-averaged methane concentration (XCH 4 ) over rice paddy-dominated regions and interannual variations in MODIS-based rice paddy areas during 2000–2015 in monsoon Asia ( a ), China ( b ), and India ( c ). The curves above are time series of monthly SCIAMACHY CH 4 column volume mixing ratios (VMRs, in parts per billion) during 2003–2009 and monthly TANSO-FTS CH 4 column VMRs during 2010–2015. The XCH 4 outliers in winter have been removed. The blue and red dashed lines are average annual values of SCIAMACHY XCH 4 and TANSO-FTS XCH 4 , respectively. The black lines and black dashed lines below indicate trends of rice paddy area for different periods in monsoon Asia, China, and India. The rice paddy-dominated regions are shown in Supplementary Fig. 35 . The linear trends and its significance levels for different periods are shown below the panels; the formulas in black color are for paddy rice planting area, and the formula in red is for XCH 4 . Source data are provided as a Source Data file. Full size image What factors drove the interannual variations of atmospheric CH 4 concentration since 2007 is still a hotly debated issue [1] , [2] , [3] , [4] , [5] , [6] , [7] , [8] , [9] , [10] , [11] , as CH 4 emissions are controlled by multiple sources and sinks. At the rice paddy fields, there are several factors which could affect its methane emission, including paddy rice planting area, cropping system, yield, management (e.g., irrigation, fertilization), and rice varieties [14] , [59] . For the first time, our study shows the fingerprint of rice paddies in the spatial distribution and seasonal dynamics of atmospheric methane concentration by using unprecedented annual paddy rice maps. We are not in position to do a full-scale (multivariate) attribution analysis on the question why atmospheric XCH 4 increased again after 2007, thus a thorough explanation of the renewed growth in XCH 4 since 2007 needs further study. Potential of annual paddy rice maps for CH 4 models To our knowledge, our annual maps of rice paddies in monsoon Asia during 2000–2015 are the first of its kind and are likely to have significant implications for simulations of biogeochemical models and atmospheric chemistry and transport models. Several empirical and process-based biogeochemical models have been used to predict CH 4 emissions from rice paddies [13] , [14] , [55] , [56] , [60] . However, most of the estimates of rice paddy CH 4 emission from those models were generally driven by rice paddy data from agricultural statistical sources such as province- or county-level administrative units [13] , [14] , [59] , [60] , [61] , which led to a large spatial uncertainty in estimates of rice paddy CH 4 emission. For example, Zhang et al. [60] estimated CH 4 emission from rice paddies at the global scale based on inundation areas, statistical data, and additional cropland masks. However, the methane emission estimates in some regions with dense rice paddies were missed due to inaccurate rice paddy distribution information, such as the northwest of Indo-Gangetic Plain in India and Pakistan. The annual maps of rice paddies at moderate spatial resolution in this study offer new opportunities to improve simulations of biogeochemical models for CH 4 emission from rice paddies. The improved estimates of CH 4 emission fluxes with high-accuracy annual paddy rice maps could then be used by atmospheric chemistry and transport models to study the spatial and seasonal consistency between atmospheric CH 4 concentration and rice paddies, as well as the relative contribution of rice paddies to the interannual dynamics of atmospheric CH 4 concentration. These new paddy rice maps will likely shed new light on the role of rice paddies in atmospheric CH 4 concentration and represent a critical step for improving the understanding of long-term dynamics of atmospheric CH 4 concentration. Agricultural emissions account for more than half of the total CH 4 emissions budget in monsoon Asia, of which one-third is estimated to originate from rice paddies [13] . Using annual paddy rice maps at 500-m spatial resolution and spaceborne XCH 4 data in monsoon Asia, this study clearly characterizes the fingerprints of rice paddies in the spatial distribution and seasonal dynamics of atmospheric CH 4 concentration over the dense rice paddy regions. It highlights an important impact of rice agriculture on the spatial and seasonal patterns of regional atmospheric CH 4 . The observed changes in the spatial distribution of rice paddies in monsoon Asia during 2000–2015 do warrant urgent and further use of the annual paddy rice maps in biogeochemical model simulations. Considering the fertilization effect of global rising atmospheric CO 2 , climate change, and projected increases in demand for rice in the coming decades, CH 4 emissions from rice production is expected to rapidly increase [15] , possibly leading to stronger effects on the variability of atmospheric CH 4 at various spatial and temporal scales. This study also provides new insight to the debates on the driving factors for the renewed growth of atmospheric CH 4 concentration since 2007 from the perspective of paddy rice planting area; and the results show the inconsistent interannual variations of rice paddy area and XCH 4 . However, considering the complexity in the CH 4 emission and atmospheric transport, more methane sources and sinks should be considered for a thorough explanation of the renewed growth of atmospheric CH 4 concentration since 2007. Atmospheric CH 4 concentration data We used the IMAP 7.1 product from SCIAMACHY [62] and the OCPR7.0 product from TANSO-FTS [63] , which were downloaded from the data portal ( http://www.esa-ghg-cci.org/sites/default/files/documents/public/documents/GHG-CCI_DATA.html ). The SCIAMACHY XCH 4 data during 2003–2011 and the TANSO-FTS XCH 4 data during 2010–2015 were arranged into 0.5° × 0.5° and 2° × 2° grids in latitude and longitude, respectively, and then composited it into monthly average XCH 4 . MODIS data We used MODIS Collection-6 surface reflectance, land surface temperature (LST), and land cover type to extract rice paddies in monsoon Asia. The 8-day composite surface reflectance products from EOS-Terra-MODIS (MOD09A1) at 500 m spatial resolution during 2000–2015 were used to calculate three spectral indices: EVI [32] , Land Surface Water Index (LSWI) [64] , and Normalized Difference Snow Index (NDSI) [65] . The bad observations containing clouds or snow were excluded before mapping rice paddies. We used the 8-day composite LST products from EOS-Aqua-MODIS (MYD11A2) at 1 km spatial resolution during 2003–2015 to determine the start and end of thermal growing season (Supplementary Fig. 21 ) and the time window of rice transplanting. The EOS-Terra-MODIS (MOD12Q1) provided wetland maps as a non-crop mask based on the land cover scheme of International Geosphere-Biosphere Programme (IGBP) (Supplementary Fig. 22 ). More detailed MODIS data processing is stated in Supplementary Note 2. Paddy rice mapping The annual maps of paddy rice in monsoon Asia at 500 m resolution from 2000–2015 were developed using time series MODIS data and a well-documented phenology-based algorithm [28] , [29] , [30] , [31] . The flooding signal during the rice transplanting phase is a critical feature used to identify rice paddies, as paddy rice is the sole crop type to be transplanted and grown in water–soil mixture fields. Through temporal profile analysis of remote sensing data, the mixture of rice plants and water (open canopy) during the transplanting phase can be tracked by the relationship between the vegetation greenness index (i.e., EVI) and the water index (i.e., LSWI) simply using the equation: LSWI + 0.05 ≥ EVI [28] , [29] . We recently improved the algorithm by incorporating the temperature-based time window for rice transplanting, which was derived from MODIS LST data [31] . We applied this method successfully in China and India in our previous study [30] . Here, the algorithm was used for monsoon Asia over the period of 2000–2015 (Supplementary Note 3). In order to improve the accuracy of the MODIS-based paddy rice mapping, several non-cropland masks were generated [28] , [29] , [30] , [31] , including evergreen vegetation, forest, sparse vegetation, natural wetlands, topographic masks, and a temperate-based mask (Supplementary Note 3, Supplementary Fig. 22 ). After excluding areas using these masks, annual paddy rice maps were generated. The resultant maps were then validated through comparing with existing products in different countries (Supplementary Note 4 and Supplementary Figs. 23 – 26 ), as well as the statistical data of FAO Statistical Databases (FAOSTAT) at national scale during 2000–2015 (Supplementary Note 4 and Supplementary Fig. 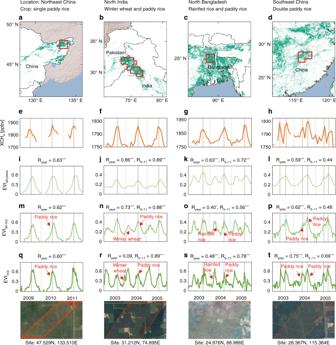27 ). We also validated the maps based on pixel-level comparison using higher resolution Landsat-based paddy rice maps in sample regions (Supplementary Note 4, Supplementary Fig. Fig. 3: Seasonal dynamics of atmospheric methane concentration and rice growth. The column-averaged methane concentration (XCH4) and the enhanced vegetation index (EVI) were analyzed in four regions of interest (ROIs) with dense rice paddies and different cropping systems.a–dSpatial distributions of rice paddies retrieved from MODIS data with 500 -m resolution in the Sanjiang Plain of Northeast China in 2010 with single cropping paddy rice (a), North India in 2005 with winter wheat and paddy rice (b), North Bangladesh in 2005 with rainfed rice and paddy rice (c), and Poyang Lake of China in 2005 with early and late paddy rice (d). The four ROIs are shown in Fig.1awith small and red polygons.e–hTime series of monthly SCIAMACHY CH4column volume mixing ratios (VMRs, in parts per billion) over the corresponding four ROIs labeled in (a–d) with red polygons.i–lTime series of monthly MODIS-based EVI for all pixels within 0.5° gridcells (EVIall-pixels) over the aforementioned four ROIs.m–pTime series of 8-day EVI values for all 500 m rice paddy pixels within the 0.5° gridcells (EVIall-rice).q–tTime series of 8-day EVI values for one rice paddy pixel with 500 m resolution (EVIrice). The four bottom images are the corresponding landscapes for each rice paddy pixel (q–t) with the extent of 500 m by 500 m from Google Earth. Ryearand R5–11offer the Pearson’s correlation coefficients between XCH4and EVI for the whole year and summer-fall season from May to November during the corresponding period labeled in thex-axis of (q–t). ***P< 0.01; *P< 0.10. Correlation coefficients without asterisk are insignificant (P> 0.10). Source data are provided as a Source Data file. 28 , and Supplementary Table 3 ). The validation and comparison results showed the continental-scale paddy rice maps were reliable. To analyze the spatial and seasonal relationships between rice paddies and satellite-observed XCH 4 , the paddy rice maps with 500 m resolution (binary map with 0 or 1) were aggregated to 0.5° and 2° gridcells with rice paddy area proportions to match the resolutions of SCIAMACHY and TANSO-FTS based XCH 4 , respectively (Supplementary Fig. 29 ). Trend analysis of rice paddy area We investigated the spatial pattern of changes in rice paddy area in monsoon Asia using the least square method. We aggregated binary paddy rice maps into fractional rice maps within 10 × 10 pixel gridcells (~5 km spatial resolution) and calculated a spatially explicit map of the linear trend of rice paddy area changes from 2000–2015 within the gridcells (Fig. 1b ). Analysis of spatial consistency between rice paddy and XCH 4 We investigated the spatial correlation between XCH 4 from SCIAMACHY/TANSO-FTS and MODIS-based rice paddy area percentage over six 3-year periods (2003–2005, 2005–2007, 2007–2009, 2009–2011, 2011–2013, and 2013–2015), forming a complete coverage in all the 3-year moving windows from 2003 to 2015 (Supplementary Fig. 30 ). The composites of six periods of observations were set considering the available years of the observed atmospheric CH 4 concentration data and the effects of potential abnormal observations in some grids and certain year. First, we analyzed variations in 3-year average yearly and seasonal XCH 4 within different rice paddy density gradients to see whether the variations of XCH 4 and rice paddy area were consistent. Then, the spatial error model (SEM) [66] was used to evaluate the correlation between XCH 4 and rice paddy area percentage in monsoon Asia, as these two variables spatially auto-correlate over geographical distribution, which would affect correlation analyses between them. Taking the data during 2003–2005 for example, we tested the spatial autocorrelation of our dependent variable (XCH 4 ) and found a significant autocorrelation, with Moran’s I equal to 0.83 ( P < 0.001) (Supplementary Table 1 ). When we used the ordinary least-squares model (OLS) to analyze the spatial relationship between XCH 4 and paddy rice croplands, the Moran’s I of model residual was 0.80 with P < 0.001 (Supplementary Table 4 ), showing the relationship did not satisfy the hypothesis of independent identical distribution and OLS was inapplicable. We then used the SEM to analyze the spatial relationship between them, and Moran’s I of model residual was −0.15 with P equal to 1 (Supplementary Table 1 ), indicating that the SEM-based result was reliable. The SEM coefficients showed that there was a significant positive correlation (all of P -value < 0.001) between spatial distributions of XCH 4 and rice paddy area percentage during the six 3-year periods (Supplementary Table 1 ). Analysis of seasonal dynamics of paddy rice growth and XCH 4 The effects of paddy rice growth on the seasonal variations of XCH 4 were examined by time series analysis of XCH 4 and MODIS-based EVI (as a proxy of rice plant growth), over four typical regions of interest (ROIs) with dense rice paddy areas and different rice cropping systems, and the rice paddy-distributed region in monsoon Asia. We also compared landscape scale EVI data and CH 4 emissions from eight existing rice paddy eddy flux sites to verify the seasonal consistency between observed CH 4 emission and rice plant growth [25] , [26] , [27] , [41] , [42] , [45] , [46] , [47] (Supplementary Fig. 14 ). Given the small size of the study plots at these flux sites, the EVI with 250 -m resolution derived from MOD13Q1 during the corresponding period was used to characterize the paddy rice growth. At the regional scale, four ROIs (Fig. 3a–d ) with different rice phenology and cropping systems were extracted from dense rice paddy gridcells with rice paddy proportions over 20% (Supplementary Fig. 31 ) to analyze the seasonal relationships between the growth of paddy rice and XCH 4 . We calculated mean EVI values from different statistical approaches: all pixels within 0.5° gridcells (EVI all-pixels ), all rice paddy pixels within 0.5° gridcells (EVI all-rice ), and single rice paddy pixel with 500 m resolution (EVI rice ). Then we analyzed the seasonal dynamics of XCH 4 and three EVI proxies in these four ROIs (Fig. 3 ), by using correlation analysis for the entire year (R year ) and summer-fall season (R 5–11 , rice growing season in the wheat–rice or other cropping system). Monsoon Asia is dominated by single- and double-cropping system [52] , [54] , [67] , [68] , and the triple-cropping is very limited in some regions like Mekong Delta [54] , [67] (Supplementary Fig. 32 ). The main growing season of rice plants in monsoon Asia are mostly during summer-fall season from May to November (Supplementary Figs. 33 , 34 ) based on statistics on the monthly distribution of rice paddy area for Asia [69] . In order to reflect the seasonal controls of paddy rice growth on atmospheric CH 4 concentration, the period of the major rice cycle (from May to November) is used to analyze the seasonal relationships between them. At the continental scale, a wall-to-wall correlation analysis was used to quantify the relationship between the seasonal variations of XCH 4 and EVI at 0.5° gridcells for the entire year (R year ) and summer-fall season (R 5–11 ) during 2003–2005 (Fig. 4 ), 2005–2007, 2007–2009, and 2009–2011 (Supplementary Figs. 17 – 19 ). The periods after 2011 were not considered due to the coarse resolution of the TANSO-FTS XCH 4 data. The region with a 3-year averaged rice paddy gridcells with area proportion larger than 10% during the corresponding period was considered here. Analysis of interannual variations of rice paddy and XCH 4 The interannual variations and trends in MODIS-based rice paddy areas and XCH 4 were analyzed to examine the potential contribution of rice paddy area dynamics to atmospheric CH 4 concentration in monsoon Asia, China, and India. The analyses were conducted from two levels: the rice paddy-dominated area (Fig. 5 ) and the whole area of monsoon Asia, China, and India (Supplementary Fig. 20 ). The rice paddy-dominated area here meant those gridcells (0.5° × 0.5°) with maximum rice paddy area proportion larger than 10% during 2000–2015 (Supplementary Fig. 35 ). Rice paddy CH 4 emission reflected by estimates of EDGAR We used the independent bottom-up estimates of Emissions Database for Global Atmospheric Research (EDGAR) data sets v4.3.2 [70] to analyze the relative contribution of rice agriculture to total CH 4 emission. The result showed that the paddy rice cultivation is the dominated sector for the CH 4 emission in the paddy rice planting area of monsoon Asia (Supplementary Fig. 36 ); specifically, the relative contribution of paddy rice cultivation CH 4 emission is >30% in the gridcells where the rice paddy area proportion is >5%. This added analysis can help us to understand the fingerprint of rice paddies in the spatial distribution and seasonal dynamics of atmospheric methane concentration in monsoon Asia. Reporting summary Further information on research design is available in the Nature Research Reporting Summary linked to this article.